Functionalization of the living diatomThalassiosira weissflogiiwith thiol moieties Biomineralization processes identified within diatoms have inspired the design of synthetic silica structures in vitro using alkoxysilane precursors. Here we explore the use of the machinery within the living diatom to fabricate organo-silica constructs using a combination of alkoxysilane and organoalkoxysilane precursors. We report on the incorporation of thiol moieties into the diatom during frustule synthesis. Formation of valves within the parent diatom is monitored using fluorescence microscopy, and the modification of the chemical composition of the diatom is confirmed using energy dispersive X-ray spectroscopy, X-ray photoelectron spectroscopy and 29 Si-nuclear magnetic resonance spectroscopy. Chemical modification is achieved without loss of the nano-scale architectural features of the frustule. Extension of this work may allow the chemistry of the diatom to be tailored during synthesis. Diatoms are unicellular algae with a hallmark intricate siliceous cell wall, known as a frustule, comprised of two valves. The exact biomineralization processes involved in the generation of the complex hierarchical architecture of the frustule are as yet unknown. However, it is known that silaffins [1] , [2] and long-chain polyamines [3] are involved in valve synthesis within a specialized unit in the parent diatom known as the silica deposition vesicle (SDV) [4] . Unravelling these mechanisms has enabled the generation of synthetic silica structures in vitro under mild conditions using synthetic silaffins and long-chain polyamines [5] , [6] , [7] . The alkoxysilane tetramethoxysilane (TMOS) has been shown to form SiO 2 in the presence of silaffins in vitro [8] following a typical sol-gel process whereby the alkoxide undergoes hydrolysis and the resulting sol gradually evolves towards the formation of a continuous colloidal network [9] . Considering the similarity between hydrolyzed TMOS and sodium silicate, the natural source of silica for diatoms, it seems reasonable that both precursors are capable of forming SiO 2 in the presence of silaffins. Condensation of organoalkoxysilanes has been reported in sol-gel science because of the wide diversity of properties that the resulting hybrid materials may offer [10] , [11] , [12] . They are typically co-condensed with alkoxysilanes to tailor the crosslinking of the resulting silica network [13] , [14] , [15] , [16] , [17] , [18] . However, co-condensation of siloxane precursors in the presence of silaffins remains under-explored and is unexplored in the living diatom. The goal of this study is to functionalize the living diatom via co-condensation of organoalkoxysilanes within the SDV of the parent diatom. For this purpose, it is hypothesized that TMOS and 3-mercaptopropyltrimethoxysilane (MPTMS) will provide a source of silica for the growth of the diatom Thalassiosira weissflogii enabling metabolic insertion of the organoalkoxysilane into the diatom frustule. The proposed mechanism of co-condensation of TMOS and MPTMS within the SDV and incorporation into the newly synthesized valve is illustrated in Fig. 1 . A 3:1 molar ratio of TMOS:MPTMS is chosen based on the observation that silica networks, prepared using regular sol-gel processes, exhibited a balance between degree of crosslinking and organic functionalization, when prepared using similar ratios [19] , [20] . In this study chemical modification of the living diatom T. weissflogii is achieved without altering the gross morphology of the frustule. 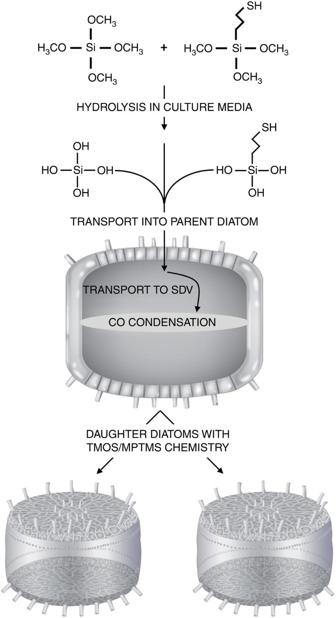Figure 1: Thiol-functionalization ofThalassiosira weissflogii. Proposed hydrolysis of TMOS/MPTMS in the culture media, transport into diatom, subsequent co-condensation within the silica deposition vesicle and incorporation into the frustule. Figure 1: Thiol-functionalization of Thalassiosira weissflogii . Proposed hydrolysis of TMOS/MPTMS in the culture media, transport into diatom, subsequent co-condensation within the silica deposition vesicle and incorporation into the frustule. Full size image T. weissflogii growth patterns TMOS and MPTMS were used in combination as it was envisaged that MPTMS could not reach a sufficient degree of crosslinking in the siloxane network to form the frustule structure in the absence of TMOS. Frustule synthesis was monitored using the fluorescent probe [2-(4-pyridyl)-5-((4-(2-dimethylaminoethylamino-carbamoyl)methoxy)phenyl)oxazole] (PDMPO) [21] , [22] , [23] as the dye is incorporated in the valves during formation ( Fig. 2a–g ). T. weissflogii cultures grown in the presence of MPTMS exhibited negligible fluorescence indicating that valve synthesis is arrested ( Fig. 2h ). Conversely, TMOS/MPTMS supported valve synthesis ( Fig. 2j ), illustrating the requirement for co-incubation of the cultures with TMOS and MPTMS. 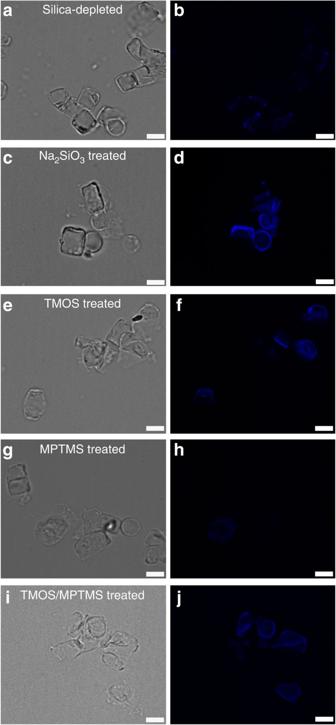Figure 2: Valve synthesis. Valve synthesis occurs whenT. weissflogiiis cultured in the presence of TMOS/MPTMS. Brightfield (a,c,e,g,i) and fluorescent (b,d,f,h,j) images ofT. weissflogiicultures grown in the presence of 100 ng ml−1PDMPO for 24 h. Valve synthesis is not observed in silica-depleted cultures or MPTMS-treated cultures. A silica precursor capable of generating a siloxane backbone is necessary for valve synthesis. Scale bar, 10 μm. Figure 2: Valve synthesis. Valve synthesis occurs when T. weissflogii is cultured in the presence of TMOS/MPTMS. Brightfield ( a , c , e , g , i ) and fluorescent ( b , d , f , h , j ) images of T. weissflogii cultures grown in the presence of 100 ng ml −1 PDMPO for 24 h. Valve synthesis is not observed in silica-depleted cultures or MPTMS-treated cultures. A silica precursor capable of generating a siloxane backbone is necessary for valve synthesis. Scale bar, 10 μm. Full size image The uptake and incorporation of TMOS/MPTMS into the frustule begins with the hydrolysis of the silanes in the culture media. As the hydrolysis of silanes leads to the release of methanol, it was critical to investigate possible detrimental effects of methanol on the growth of T. weissflogii. The concentration of methanol investigated was based on a theoretical value of methanol released from TMOS:MPTMS, at a 3:1 molar ratio, as shown in equation 1. It was determined that 1 mM methanol does not inhibit growth of T. weissflogii ( Supplementary Fig. S1 ). In addition, it was necessary to establish the growth profile of T. weissflogii in silica-depleted media to serve as a control when investigating growth patterns in the presence of a silica precursor. The growth patterns of silica-depleted cultures exhibited a significant reduction in growth after 48 h when compared with silica-treated cultures ( Supplementary Fig. S1 ). 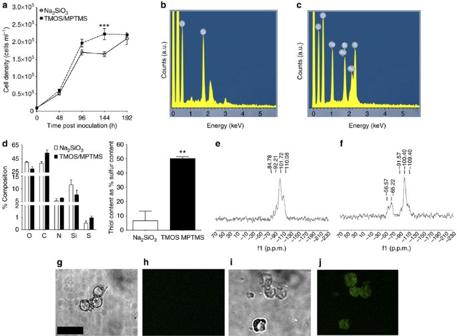Figure 3: Modification ofT. weissflogiiwith TMOS/MPTMS. (a) The growth profile ofT. weissflogiigrown in the presence of Na2SiO3or TMOS/MPTMS added at 48 h intervals. Two-way analysis of variance followed by Bonferronipost hocanalysis revealed statistical difference at 144 h ***P<0.001. Data expressed as mean±s.e.m. (n=6). SEM–EDX spectra of (b)T. weissflogiiand (c) TMOS/MPTMST. weissflogiishow presence of a sulphur peak in the latter only. (d) Elemental composition ofT. weissflogiiand TMOS/MPTMST. weissflogiidetermined by XPS analysis.t-test revealed that the thiol content is significantly higher in TMOS/MPTMST. weissflogii. Data are presented as mean±s.e.m.(n=3) **P<0.05.29Si-NMR spectra of (e)T. weissflogiiand (f) TMOS/MPTMST. weissflogiishow the characteristic peaks due to Si–O and Si–Si bonds. Peaks due to organo-Si bonds are present in the latter only. Fluorescent labelling of the thiol moiety with SBDF on cleaned frustules revealed an absence of the functional group onT. weissflogiiand its presence on TMOS/MPTMST. weissflogii. Brightfield and fluorescent images of (gandh) unmodified and (iandj) modifiedT. weissflogii. Scale bar, 20 μm. Figure 3a shows the growth profile of TMOS/MPTMS-treated cultures. The absence of a reduction in growth after 48 h indicates that the cultures did not experience silica depletion. Furthermore, the profile is similar to sodium metasilicate non-hydrate (Na 2 SiO 3 )-treated cultures. This evidence supports the hypothesis that TMOS/MPTMS serves as a source of silica for growth of T. weissflogii . Figure 3: Modification of T. weissflogii with TMOS/MPTMS. ( a ) The growth profile of T. weissflogii grown in the presence of Na 2 SiO 3 or TMOS/MPTMS added at 48 h intervals. Two-way analysis of variance followed by Bonferroni post hoc analysis revealed statistical difference at 144 h *** P <0.001. Data expressed as mean±s.e.m. ( n =6). SEM–EDX spectra of ( b ) T. weissflogii and ( c ) TMOS/MPTMS T. weissflogii show presence of a sulphur peak in the latter only. ( d ) Elemental composition of T. weissflogii and TMOS/MPTMS T. weissflogii determined by XPS analysis. t -test revealed that the thiol content is significantly higher in TMOS/MPTMS T. weissflogii . Data are presented as mean±s.e.m. (n =3) ** P <0.05. 29 Si-NMR spectra of ( e ) T. weissflogii and ( f ) TMOS/MPTMS T. weissflogii show the characteristic peaks due to Si–O and Si–Si bonds. Peaks due to organo-Si bonds are present in the latter only. Fluorescent labelling of the thiol moiety with SBDF on cleaned frustules revealed an absence of the functional group on T. weissflogii and its presence on TMOS/MPTMS T. weissflogii . Brightfield and fluorescent images of ( g and h ) unmodified and ( i and j ) modified T. weissflogii . Scale bar, 20 μm. Full size image Chemical characterization of TMOS/MPTMS T. weissflogii The chemical composition and architectural features of TMOS/MPTMS T. weissflogii were characterized extensively. Scanning electron microscopy–energy dispersive X-ray spectroscopy (SEM–EDX) analysis confirmed the absence of a sulphur peak in T. weissflogii ( Fig. 3b ) and the presence of one in the TMOS/MPTMS-modified diatom ( Fig. 3c ). This was corroborated by EDX-transmission electron microscopy analysis ( Supplementary Fig. S2a ). X-ray photoelectron spectroscopy (XPS) analysis of elemental composition revealed that TMOS/MPTMS T. weissflogii had an increase in sulphur and carbon content and a decrease in silica content compared with T. weissflogii ( Fig. 3d ). The sulphur species present in TMOS/MPTMS T. weissflogii were predominantly thiol moieties, contributing to 51±1.4% of the sulphur content. The 29 Si-CP MAS NMR spectrum of TMOS/MPTMS-modified diatoms showed two groups of chemical shifts ( Fig. 3f ); T units (T2 and T3 at −56.5 and −65.2 p.p.m., respectively) and Q units (Q2, Q3 and Q4 at −91.6, −100.4 and −109.4 p.p.m., respectively). The qualitative pattern of Q units obtained from CP MAS NMR was typical of amorphous silica and was similar to both that of T. weissflogii ( Fig. 3e ) and that reported for different diatom species [24] . In comparison to T. weissflogii , the presence of T2 and T3 units in TMOS/MPTMS-modified diatoms confirmed the presence of an organic moiety pending from the Si backbone of the hybrid diatoms skeleton. This feature was confirmed by the pattern of Q units obtained from the 29 Si-MAS NMR of TMOS/MPTMS-modified diatoms ( Supplementary Fig. S2b ), with an increase of the intensity ratio between Q3 and Q4 units as compared with that previously reported [24] . Fluorescent labelling of the cleaned diatoms with a thiol specific probe confirmed the absence of thiol moieties on T. weissflogii ( Fig. 3g,h ) and presence of thiol moieties on the surface of TMOS/MPTMS T. weissflogii ( Fig. 3i,j ). Architectural characterization of TMOS/MPTMS T. weissflogii The native T. weissflogii has characteristic fultoportulae that decorate the edge and the centre of the diatom ( Fig. 4a ). Ribs radiate from the centre to the periphery of the diatom, and the valve face is decorated with pores ( Fig. 4b,c ). The gross morphology of the TMOS/MPTMS-modified diatom is unaltered ( Fig. 4d–f ). Atomic force microscopy (AFM) analysis revealed that the distance between ribs in both a radial and a rotational direction is decreased in TMOS/MPTMS T. weissflogii ( Fig. 4g ). Significant reductions in the pore dimension of the TMOS/MPTMS-modified diatom ( Fig. 4h ) were seen. The alterations in the pore parameters may be attributed to changes in the siloxane backbone of the frustule following the incorporation of the thiol moieties ( Supplementary Fig. S3 ). The decreased density of silica in TMOS/MPTMS T. weissflogii could lead to a less compact frustule and subsequent reductions in pore parameters. No reduction in the number of pores per unit area is observed ( Fig. 3i ). 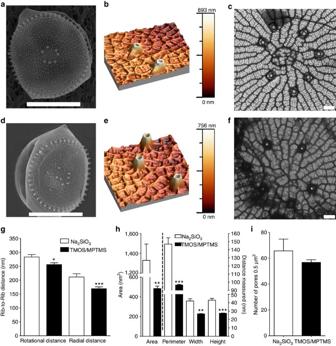Figure 4: TMOS/MPTMST. weissflogiiretains nano-scale architectural features. SEM micrographs of (a)T. weissflogiiand (d) TMOS/MPTMST. weissflogii. Scale bar, 10 μm. Surface topography of the valve surface of (b)T. weissflogiiand (e) TMOS/MPTMST. weissflogiiimaged using AFM illustrating the characteristic features in the centre of the valve. TEM micrographs of (c)T. weissflogiiand (f) TMOS/MPTMST. weissflogiiillustrating the decreased pore parameters in the modified diatom. Scale bar, 500 nm (g) Distance between ribs is decreased in TMOS/MPTMST. weissflogii. Data are shown as mean±s.e.m. (Rotational distancen⩾75 measurements, Radial distancen⩾35 measurements)t-test revealed significant difference between groups *P<0.05, ***P<0.001. (h) Architectural properties of the pores on the valve surface are reduced in TMOS/MPTMST. weissflogii. Data represent mean±s.e.m. (n=3)t-test revealed significant difference between groups **P<0.005, ***P<0.001 (i) The density of pores on the valve surface is unaltered. Data represent mean±s.e.m. (n=3). Figure 4: TMOS/MPTMS T. weissflogii retains nano-scale architectural features. SEM micrographs of ( a ) T. weissflogii and ( d ) TMOS/MPTMS T. weissflogii . Scale bar, 10 μm. Surface topography of the valve surface of ( b ) T. weissflogii and ( e ) TMOS/MPTMS T. weissflogii imaged using AFM illustrating the characteristic features in the centre of the valve. TEM micrographs of ( c ) T. weissflogii and ( f ) TMOS/MPTMS T. weissflogii illustrating the decreased pore parameters in the modified diatom. Scale bar, 500 nm ( g ) Distance between ribs is decreased in TMOS/MPTMS T. weissflogii . Data are shown as mean±s.e.m. (Rotational distance n ⩾ 75 measurements, Radial distance n ⩾ 35 measurements) t -test revealed significant difference between groups * P <0.05, *** P <0.001. ( h ) Architectural properties of the pores on the valve surface are reduced in TMOS/MPTMS T. weissflogii . Data represent mean±s.e.m. ( n =3) t -test revealed significant difference between groups ** P <0.005, *** P <0.001 ( i ) The density of pores on the valve surface is unaltered. Data represent mean±s.e.m. ( n =3). Full size image Previous studies have explored FITC-labelled silanes to explore valve formation in T. weissflogii [25] ; however, this is the first study to demonstrate that organoalkoxysilanes can be used as a source of silica for growth of the diatom. The incorporation of MPTMS into the frustule was confirmed by SEM-EDX, XPS, Si-NMR, and TEM–EDX analyses. The thiol moiety has a functional role and has been used in studies to demonstrate removal of heavy metals from water samples [26] , [27] . The possibility of using the living diatom following modification of the chemistry of the frustule is an exciting area of research. The results of this study open avenues for further investigations to alter the chemistry of living silicaceous organisms using organoalkoxysilanes. Materials TMOS, MPTMS, sodium metasilicate non-hydrate, 7-fluorobenzo-2-oxa-1,3-diazole-4-sulphonic acid ammonium (SBDF), dimethylsulphoxide, methanol, buffer reagents and artificial seawater (ASW) reagents were purchased from Sigma Aldrich (Ireland). Lysosensor Yellow/blue DND-160 (PDMPO) was purchased fromInvitrogen (France). Cultivation of T. weissflogii T. weissflogii , isolated from Galway Bay, Ireland, was grown in ASW, prepared according to Berges et al . [28] enriched with Guillard’s f/2 marine enrichment media without silicates, at a 14-h:10-h light:dark cycle, light intensity of 3,000 lux and temperature range of 16–22°C. Cultures were grown in polystyrene tissue culture flasks. Preparation of modified T. weissflogii T. weissflogii was inoculated in silicate-free-enriched ASW for a minimum 24 h. Starved cultures were centrifuged at 2,500 g for 20 min and washed with silicate-free ASW three times. Fresh cultures were inoculated at a cell density of 1 × 10 4 cells ml −1 in a total volume of 200 ml enriched-ASW. TMOS/MPTMS (3:1) or Na 2 SiO 3 was added to cultures at a final concentration of 200 μM Si at time of inoculation and at 48 h intervals ( Supplementary Fig. S4 ). Cultures were collected 192 h post inoculation and cleaned as detailed below. The diatom cell density was monitored using a haemocytometer. Visualization of valve synthesis using PDMPO Starved T. weissflogii cultures were inoculated at a cell density of 1 × 10 4 cells ml −1 . Na 2 SiO 3 , TMOS, MPTMS or TMOS/MPTMS (3:1) was added to cultures at a final concentration of 200 μM Si at time of inoculation. PDMPO was added to cultures at a final concentration of 100 ng ml −1 . Diatom cultures were grown for 24 h. Cleaned frustules were allowed to air dry on a glass slide. Images were captured as Z-Stacks on an Andor Olympus Spinning Disk Microscope (Andor, Belfast, Northern Ireland), using Andor IQ software, with a × 60 oil immersion objective lens—NA 1.42. Before collecting the Z-stack, exposure time and electron multiplying gain were set and recorded to the channel of illumination. The specimen was imaged using a λ405-nm (Blue-Violet) laser to produce blue fluorescence. Images were taken at 0.25 μm apart. Preparation of cleaned frustules for characterization Organic matter was removed from the diatoms by successive washes with heated de-ionized water (60°C), de-ionized water and methanol. Diatoms were suspended in heated de-ionized water for 20 min followed by centrifugation at 2,500 g for 20 min. This was repeated three times. Three washes in de-ionized water followed. The final cleaning step involved a minimum of three washes in methanol until the pellet appeared white in colour. Cleaned frustules were examined by SEM–EDX, TEM–EDX, XPS, 29 Si-NMR and AFM analysis. Characterization of frustules by SEM–EDX Cleaned frustules suspended in methanol were allowed to air dry on a carbon stub and were subsequently gold coated. SEM–EDX analysis was performed using Hitachi S-4700 SEM with INCA software (Oxford Instruments). Frustules were analysed on valve faces that were clearly visible. Characterization of frustules by TEM Cleaned frustules suspended in methanol were allowed to air dry on a copper grid. TEM-EDX analysis was performed with a JEOL 2100F operated at 200 kV using a field emission electron source equipped with a Gatan Ultrascan Camera. The identity of each element was confirmed using an EDAX detector and Genesis software. Characterization of the pore parameters and pore distribution was performed using ImageJ software on TEM images collected using Hitachi H-7500 TEM with AMT image capture software. t -tests were performed to determine differences between treatment groups. Characterization of frustules by XPS Cleaned frustules were dried at 60 °C for 48 h. Samples were dusted onto a double-sided adhesive and analysed using Kratos AXIS -165 spectrometer using monochromatic Al Kα radiation. XPS analyses were calibrated with respect to the carbon 1s excitation (284.8 eV). Characterization of frustules by 29 Si-NMR The 29 Si-CP MAS solid state NMR spectra of clean dried frustules were acquired at room temperature using a BRUKER AV-400-WB using a 4-mm BRUKER probe of ZrO mounted with a stopper of Kel-F. The working frequencies were 79.5 and 400.1 MHz for 29 Si and 1 H NMR, respectively. The spinning frequency was 10 kHz. The pulse sequence for 1 H- 29 Si cross-polarization was composed of a π /6 pulse at 30 kHz of spectral width, 6 ms of contact time, 5 s of relaxation time and 1 H uncoupling tppm15 type at 80 KHz. The number of scans ranged from 2,048 to 9,000 depending on the sample. The chemical shift was referred to TMS (at 0 p.p.m., as primary reference) and kaolin (at −91.2 p.p.m., as secondary reference). These references were also used for the set-up of the Hartmann–Hahn operation conditions. Characterization of frustules by AFM AFM measurements were performed under ambient conditions in intermittent contact mode using a NanoWizard-II AFM coupled with an inverted optical microscope. Silicon cantilevers (spring constant, k ~2.8 N m −1 and resonance frequency, f ~75 kHz) with high aspect ratio (1:10 aspect ratio, tip radius <3 nm), high density, diamond-like carbon tips were used (MSS-FMR-13, Nanotools, Germany). Analysis of AFM images was performed using WSxM Software [29] . Fluorescent labelling of incorporated thiol moieties Thiol moieties were fluorescently labelled by incubation of cleaned frustules with 7-fluorobenzo-2-oxa-1,3-diazole-4-sulphonic acid ammonium in 0.1 M borate buffer containing 1 mM EDTA pH 9.5 for 1 h at 60 °C. Frustules were washed five times with de-ionized water before visualization ( Supplementary Fig. S5 ) using a Zeiss LSM 510 multi-photon confocal microscope. The Ti Sapphire 2-photon laser was operated at 5 W, 75% power and 780 nm. Images were collected using FITC filter. How to cite this article: Lang, Y. et al . Functionalization of the living diatom Thalassiosira weissflogii with thiol moieties. Nat. Commun. 4:2683 doi: 10.1038/ncomms3683 (2013).